The intracellular redox protein MICAL-1 regulates the development of hippocampal mossy fibre connections Mical is a reduction–oxidation (redox) enzyme that functions as an unusual F-actin disassembly factor during Drosophila development. Although three Molecule interacting with CasL (MICAL) proteins exist in vertebrate species, their mechanism of action remains poorly defined and their role in vivo unknown. Here, we report that vertebrate MICAL-1 regulates the targeting of secretory vesicles containing immunoglobulin superfamily cell adhesion molecules (IgCAMs) to the neuronal growth cone membrane through its ability to control the actin cytoskeleton using redox chemistry, thereby maintaining appropriate IgCAM cell surface levels. This precise regulation of IgCAMs by MICAL-1 is essential for the lamina-specific targeting of mossy fibre axons onto CA3 pyramidal neurons in the developing mouse hippocampus in vivo . These findings reveal the first in vivo role for a vertebrate MICAL protein, expand the repertoire of cellular functions controlled through MICAL-mediated effects on the cytoskeleton, and provide insights into the poorly characterized mechanisms underlying neuronal protein cell surface expression and lamina-specific axonal targeting. In many regions of the nervous system, afferent axon projections confine their terminal arbours and synapses to specific laminae. This facilitates the selection of appropriate postsynaptic partners and guides the formation of synaptic contacts to specific subcellular domains. Although the assembly of lamina-restricted connections is known to depend on specific extracellular cues [1] , [2] , [3] , our understanding of the intracellular mechanisms underlying this process is still limited. The hippocampus is an excellent model for studying lamina-specific connectivity because afferent projections from various brain regions terminate at specific laminae in this structure. This is exemplified by mossy fibre axons that connect dentate gyrus (DG) and CA3 neurons. Mossy fibre axons emanate from DG granule cells and are confined to two laminae on either side of the CA3 pyramidal cell layer. Mossy fibres in the stratum lucidum (SL) form the suprapyramidal bundle (SPB) and innervate the proximal-most part of the apical dendrites of CA3 pyramidal neurons, while those in the stratum oriens (SO) run in the infrapyramidal bundle (IPB) and make synaptic contacts with the basal dendrites of CA3 neurons [4] . Hippocampal mossy fibres mediate hippocampal learning and are linked to various neural disorders [5] , but the molecular mechanisms that dictate their laminar distribution remain incompletely understood. Current evidence implicates two families of extrinsic factors in directing the lamina-restricted projection of mossy fibres: plexins and immunoglobulin superfamily cell adhesion molecules (IgCAMs) [6] , [7] . Class A plexins interact in cis and/or trans with their semaphorin ligands to confine mossy fibres to the SL [8] , [9] , [10] . The precise molecular interactions underlying the IgCAM-dependent effects are less well-understood [11] , [12] , but recent work shows that tight control of IgCAM cell surface levels is essential to ensure mossy fibre lamination [13] . This observation is consistent with findings in other layered structures where spatiotemporal regulation of cell surface protein expression dictates lamina-specific connectivity [14] , [15] . Protein expression at the growth cone membrane is controlled through different mechanisms, including proteolysis, endocytosis and directed trafficking of new proteins. Although progress has been made in dissecting the role of some of these mechanisms, others, including the regulation of protein transport, remain poorly understood [16] , [17] , [18] , [19] . Here we establish a role for Molecule interacting with CasL (MICAL)-1 in the development of lamina-specific hippocampal connectivity. MICALs comprise a family of unusual intracellular proteins that catalyse reduction–oxidation (redox) reactions through their flavoprotein monooxygenase (MO) domain to regulate F-actin dynamics [20] , [21] , [22] , [23] , [24] , [25] , [26] , [27] . Although three MICALs exist in vertebrate species (MICAL-1-3), in vivo functions of MICALs have only been addressed in Drosophila , revealing roles in axon guidance, myofilament organization, dendritic pruning and bristle development [22] , [23] , [28] , [29] . Our data reveal a previously uncharacterized function for MICALs by showing that MICAL-1 controls the growth cone membrane targeting of cell adhesion molecules (IgCAMs), through redox regulation of the actin cytoskeleton. This novel molecular mechanism dictates IgCAM cell surface levels and, as a result, the function of IgCAMs in the development of lamina-specific mossy fibre connections in the postnatal hippocampus. These findings for the first time establish an in vivo function for a vertebrate MICAL protein, show that redox regulation of the cytoskeleton by MICALs functions beyond axon and cell repulsion, and provide insights into the mechanisms that dictate neuronal protein cell surface expression and lamina-specific axonal targeting. MICAL-1 expression in DG granule cells and mossy fibres Expression of MICAL-1 in the mouse postnatal hippocampus [30] led us to explore a role for MICAL-1 during hippocampal development. First, we determined the hippocampal distribution of MICAL-1 at postnatal and adult stages by immunohistochemistry. MICAL-1 was found in the DG, the polymorphic layer, and cornu ammonis (CA)1–3 ( Fig. 1a–c ; Supplementary Fig. 1 ). Notably, at P5, MICAL-1 expression was prominent in the molecular layer (ML) of the DG and in the SL. The SL is the proximal-most lamina of the suprapyramidal region of CA3 and contains mossy fibre axons of DG granule cells. The presence of MICAL-1 in postnatal mossy fibres was confirmed by immunocytochemistry of cultured DG granule cells. MICAL-1 expression was observed in the mossy fibre axons and growth cones of P7 DG neurons cultured for 3 or 7 days in vitro (DIV; Fig. 1d ). In the adult hippocampus, MICAL-1 was strongly expressed in CA3 pyramidal neurons and, at lower levels, in the DG, polymorphic layer and CA1. No specific signals were found in sections derived from MICAL-1 −/− mice ( Fig. 1c ). Thus, at postnatal stages, MICAL-1 is predominantly expressed in DG neurons and their efferent mossy fibres. 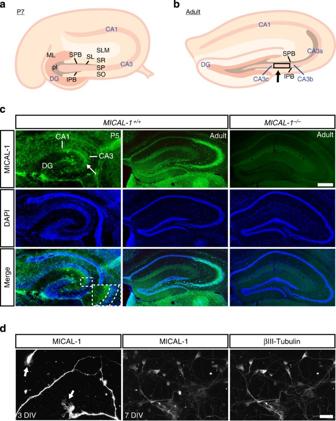Figure 1: MICAL-1 is expressed in DG granule cells, their mossy fibre projections and postsynaptic partners. (a,b) Schematic representation of the postnatal and adult mouse hippocampus. Rectangle and arrow indicate the area and location used for quantification of mossy fibre density and CA3 width, respectively. pl, polymorphic layer; SLM, stratum lacunosum-moleculare; SO, stratum oriens; SP, stratum pyramidale; SR, stratum radiatum. (c) Coronal sections immunostained for MICAL-1 (green) and counterstained with DAPI (blue). White arrow indicates MICAL-1 expression in the SL. Insert shows higher magnification of the boxed area in the lower left panel. Dashed lines in insert mark SP. Scale bar, 225 μm (P5), 150 μm (insert at P5), 400 μm (adult mutant), 450 μm (adult WT). (d) Representative images showing immunostaining for MICAL-1 in dissociated cultures of P7 DG granule cells at 3 and 7 DIV. Arrows indicate growth cones. Two right panels show co-immunostaining for MICAL-1 and βIII-tubulin. Immunostainings were repeated three times with similar results. Scale bar, 120 μm. Figure 1: MICAL-1 is expressed in DG granule cells, their mossy fibre projections and postsynaptic partners. ( a , b ) Schematic representation of the postnatal and adult mouse hippocampus. Rectangle and arrow indicate the area and location used for quantification of mossy fibre density and CA3 width, respectively. pl, polymorphic layer; SLM, stratum lacunosum-moleculare; SO, stratum oriens; SP, stratum pyramidale; SR, stratum radiatum. ( c ) Coronal sections immunostained for MICAL-1 (green) and counterstained with DAPI (blue). White arrow indicates MICAL-1 expression in the SL. Insert shows higher magnification of the boxed area in the lower left panel. Dashed lines in insert mark SP. Scale bar, 225 μm (P5), 150 μm (insert at P5), 400 μm (adult mutant), 450 μm (adult WT). ( d ) Representative images showing immunostaining for MICAL-1 in dissociated cultures of P7 DG granule cells at 3 and 7 DIV. Arrows indicate growth cones. Two right panels show co-immunostaining for MICAL-1 and βIII-tubulin. Immunostainings were repeated three times with similar results. Scale bar, 120 μm. Full size image MICAL-1 controls lamina-restricted mossy fibre projections Mossy fibre projections in the rodent hippocampus mostly develop postnatally (P0–P14) [31] . This phase of hippocampal development coincides with expression of MICAL-1 in DG granule cells and axons ( Fig. 1 ). To assess whether MICAL-1 is required for mossy fibre pathway development, we generated a conditional MICAL-1 -null mouse ( MICAL-1 f/f ; Supplementary Fig. 2 ). First, full knockout ( MICAL-1 −/− ) mice were obtained ( Supplementary Fig. 2 ). Homozygous animals were born at the expected Mendelian frequency and did not show any gross abnormalities. To visualize DG granule cells and mossy fibre axons, we performed immunohistochemistry for calbindin (CB) at P30, when mossy fibre pathfinding has been completed. In wild-type (WT) controls, CB + mossy fibres emanating from the DG bifurcated and segregated into a large SPB and IPB, respectively on either side of the stratum pyramidale (SP) of CA3, the layer containing pyramidal neuron somata. The majority of mossy fibres in the IPB ran below CA3 to join the SPB in the distal part of CA3 and only few fine IPB collaterals were observed to cross the SP before this point ( Fig. 2a ). In MICAL-1 −/− mutants, this characteristic lamination pattern was altered. At rostral levels, mossy fibres failed to bifurcate and prematurely invaded the SP, forming thick, fasciculated bundles that aberrantly navigated between CA3 somata. More caudally, the SPB was discernable in most MICAL-1 −/− mice, although it appeared less compact and reduced in width, especially in CA3c. In contrast, the IPB was absent or misplaced in the SP of MICAL-1 −/− mice ( Fig. 2a ). Quantification of CB + mossy fibre density in the SP of CA3 revealed an increase in MICAL-1 −/− mice (+/+ 100±7.0%, −/− 246±4.2%; n =6 each, P <0.01; unpaired t -test). In addition, the length of both the SPB and IPB and the distance between the SPB and IPB were decreased in MICAL-1 −/− mice ( Fig. 2b ; P <0.05; unpaired t -test). These results show that MICAL-1 is required for the lamina-restricted projection of mossy fibres, especially those forming the IPB. 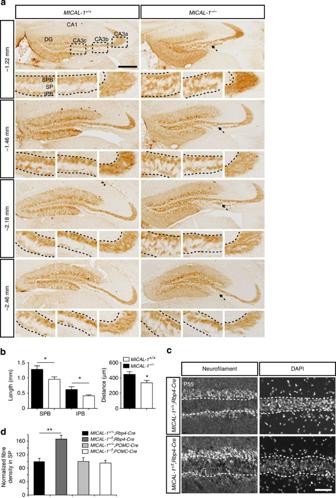Figure 2: MICAL-1 is required in DG granule cells for the lamina-specific organization of hippocampal mossy fibre projections. (a) Immunohistochemistry for CB to visualize DG granule cells and mossy fibre projections in coronal sections of P30MICAL-1+/+andMICAL-1−/−littermates at different rostral–caudal levels (numbers are corresponding anterior–posterior coordinates from bregma). Insets show higher magnifications of CA3c, b and a. Dotted lines mark the area normally covered by the stratum pyramidale (SP) and the SPB and IPB, respectively. Black arrows indicate mossy fibre misrouting into SP. Scale bar, 225 μm (inserts), 450 μm (overview). (b) Quantification of the length (left panel) and distance between (right panel) the SPB and IPB in six adultMICAL-1+/+and sixMICAL-1−/−mice. Unpairedt-test, *P<0.05. Data are presented as means±s.e.m. (c) Immunohistochemistry for NF and DAPI staining in coronal sections of P55MICAL-1+/+;Rbp4-CreorMICAL-1−/f;Rbp4-Cremice. Scale bar, 140 μm. (d) Quantification of the aberrant innervation of the SP by NF-positive mossy fibres. One-way ANOVA, **P<0.01.n=6 per group. Data are presented as means±s.e.m. Figure 2: MICAL-1 is required in DG granule cells for the lamina-specific organization of hippocampal mossy fibre projections. ( a ) Immunohistochemistry for CB to visualize DG granule cells and mossy fibre projections in coronal sections of P30 MICAL-1 +/+ and MICAL-1 −/− littermates at different rostral–caudal levels (numbers are corresponding anterior–posterior coordinates from bregma). Insets show higher magnifications of CA3c, b and a. Dotted lines mark the area normally covered by the stratum pyramidale (SP) and the SPB and IPB, respectively. Black arrows indicate mossy fibre misrouting into SP. Scale bar, 225 μm (inserts), 450 μm (overview). ( b ) Quantification of the length (left panel) and distance between (right panel) the SPB and IPB in six adult MICAL-1 +/+ and six MICAL-1 −/− mice. Unpaired t -test, * P <0.05. Data are presented as means±s.e.m. ( c ) Immunohistochemistry for NF and DAPI staining in coronal sections of P55 MICAL-1 +/+ ; Rbp4-Cre or MICAL-1 −/f ; Rbp4-Cre mice. Scale bar, 140 μm. ( d ) Quantification of the aberrant innervation of the SP by NF-positive mossy fibres. One-way ANOVA, ** P <0.01. n =6 per group. Data are presented as means±s.e.m. Full size image MICAL-1 is required in DG neurons for mossy fibre development In rats, innervation of CA3 by mossy fibres begins during early postnatal development and reaches its mature configuration around P14 (except for IPB pruning that is finalized by P45). Initially, mossy fibres are only observed in the SPB, but by P6–9, mossy fibres start to form the IPB [31] . To determine the ontogeny of the defects found in MICAL-1 mutants, coronal sections of the hippocampus of MICAL-1 +/+ and MICAL-1 −/− mice were immunostained for neurofilament (NF), to visualize mossy fibres [11] and counterstained with Nissl. Although initially the organization of the SPB and SP was intact (P0–P5), this analysis revealed numerous axons that penetrated the SP in between dispersed CA3 neurons in MICAL-1 −/− mice from P7 onwards. Quantification confirmed this aberrant pattern of mossy fibre innervation ( Supplementary Fig. 3a,b ; n =5 per stage, P <0.05, P <0.01; one-way analysis of variance (ANOVA)). During the period of mossy fibre pathfinding, hippocampal expression of MICAL-1 is most prominent in DG granule cells and their axonal projections ( Fig. 1 ). Therefore, we asked whether or not MICAL-1 is required in DG granule cells to enforce lamina-restricted distribution of their axons. We selectively ablated MICAL-1 from DG granule cells by crossing MICAL-1 f/f mice with retinol binding protein 4 (Rbp4)-Cre mice. Crossing Rbp4-Cre bacterial artificial chromosome (BAC) mice with ROSA26;eYFP reporter mice ( Supplementary Table 1 ) revealed robust Cre-loxP recombination in ~60% of DG granule cells at P4 and at P15—throughout the period of mossy fibre pathfinding ( Supplementary Fig. 4a ). No YFP signals were detected in CA3 neurons or in other parts of the postnatal hippocampus. Immunohistochemistry for NF in combination with DAPI staining revealed that CA3 neurons were dispersed and mossy fibres misguided into the SP of CA3 in P55 MICAL-1 −/f ; Rbp4-Cre mice, as compared with MICAL-1 +/+ ; Rbp4-Cre controls. DG cytoarchitecture, however, appeared normal in these mutants. These defects appeared slightly less robust compared with those observed in MICAL-1 −/− mice ( Fig. 2a ), perhaps owing to the fact that Rbp4-Cre drives Cre excision in a subset of DG granule cells ( Supplementary Fig. 4a ). No defects were observed in MICAL-1 f/f or MICAL-1 +/f ; Rbp4-Cre mice ( Fig. 2c,d ; n =6 per genotype; P <0.01; one-way ANOVA). These results show that MICAL-1 is required in DG granule cells to control the lamina-restricted organization of mossy fibres in CA3. The DG is one of the few regions of the brain where newly generated neurons are functionally incorporated at late postnatal and adult stages. To adress whether MICAL-1 contributes to the lamina-restricted wiring of mossy projections at later stages, we generated MICAL-1 −/f ; proopiomelanocortin ( POMC)-Cre mice. In the hippocampus of POMC-Cre BAC mice, Cre-loxP recombination begins between postnatal weeks 2–3 in newly born DG granule cells, which is after completion of developmental mossy fibre pathfinding ( Supplementary Fig. 4a ). No obvious defects in mossy fibre projections or CA3 layering were found in P55 MICAL-1 −/f ; POMC-Cre mice ( Fig. 2d ; Supplementary Fig. 4b ). Thus, the role of MICAL-1 in sculpting lamina-specific mossy fibre projections is restricted to early postnatal development, a result in line with the lack of MICAL-1 protein in mature mossy fibre projections ( Fig. 1 ). MICAL-1 dictates subcellular synaptic specificity in CA3 Lamina-specific axonal targeting faciliates the formation of synapses at specific subcellular domains of partner neurons. Mossy fibres in the SPB and IPB synapse on the poximal most parts of the apical and basal dendrites of CA3 pyramidal neurons, respectively. Therefore, we next examined the synaptic fate of misrouted mossy fibre terminals using Timm staining, which labels mossy fibres and their synapses. In adult WT mice, mossy fibres formed synapses with the apical and basal dendrites of CA3 pyramidal cells and only few mossy fibre synapses were present in the SP. This laminar distribution of synapses was altered in MICAL-1 −/− mice in which we observed abnormal Timm staining in the SP and disruption of the SPB and IPB ( Supplementary Fig. 4c ). This was confirmed by labelling mossy fibres and synapses separately using immunohistochemistry for NF and synaptophysin. NF + mossy fibres invaded the SP in MICAL-1 −/− mice giving rise to synaptophysin + synaptic terminals surrounding CA3 somata ( Fig. 3a ). Thus, MICAL-1 deficiency leads to the formation of ectopic synapes in the layer containing CA3 pyramidal neuron somata. 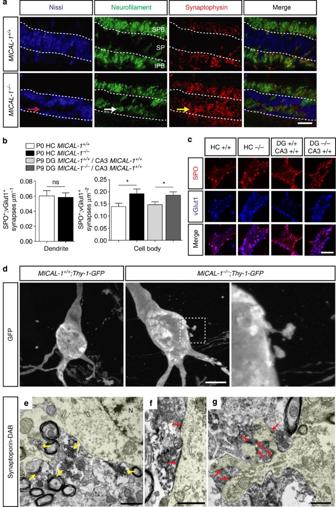Figure 3: MICAL-1 controls the subcellular site-specific distribution of mossy fibre synapses. (a) Co-immunohistochemistry for NF and synaptophysin, to label mossy fibre axons and synapses, respectively, in the CA3 region of adultMICAL-1+/+andMICAL-1−/−mice (n=3 and 3). Arrows indicate the disrupted stratum pyramidale (red; SP, dotted lines), ectopic mossy fibre projections (white) and synapses (yellow). Scale bar, 90 μm. (b) Quantification of the number of SPO+;vGlut1+mossy fibre synapses on the proximal dendrites and cell bodies ofMICAL-1+/+orMICAL-1−/−CA3 pyramidal neurons of culture experiments as shown inc.n>30 neurons per group of >3 independent cultures per genotype, from four to five different litters. Unpairedt-test, *P<0.05. Data are presented as means±s.e.m. (c) Dissociated P0–1 hippocampal cultures (HC) or co-cultures of P9 DG and CA3 neurons were fixed at 21 DIV and immunostained for SPO (red), vGlut1 (blue), CAMKII (not shown), Prox1 (not shown) and CTIP2 (not shown). Images show cell bodies of Prox1−;CTIP2−CA3 pyramidal neurons. Mossy fibre synapses appear purple. Scale bar, 10 μm. (d) Multiple large, complex spines are extending from the somata of CA3 pyramidal neurons in adultMICAL-1−/−;Thy1-GFPmice. Panel at the right shows higher magnification of boxed area in middle panel. Scale bar, 10 μm. (e–g) Immunoelectron micrographs of the SP of CA3 in SPO–DAB-stained sections from the hippocampus of adultMICAL-1−/−mice. (e) SPO+mossy fibre terminals containing numerous synaptic vesicles (yellow arrows) are located around a CA3 pyramidal neuron cell body (outlined in light yellow). (f) SPO+terminals form synapse-like junctions on a CA3 pyramidal neuron cell body (outlined in light yellow). Red arrows point to postsynaptic densities. (g) SPO+mossy fibre terminals contact a large and complex spine-like structure emanating from a CA3 pyramidal neuron cell body (outlined in light yellow). N, nucleus. Scale bars, 1 μm. Figure 3: MICAL-1 controls the subcellular site-specific distribution of mossy fibre synapses. ( a ) Co-immunohistochemistry for NF and synaptophysin, to label mossy fibre axons and synapses, respectively, in the CA3 region of adult MICAL-1 +/+ and MICAL-1 −/− mice ( n =3 and 3). Arrows indicate the disrupted stratum pyramidale (red; SP, dotted lines), ectopic mossy fibre projections (white) and synapses (yellow). Scale bar, 90 μm. ( b ) Quantification of the number of SPO + ;vGlut1 + mossy fibre synapses on the proximal dendrites and cell bodies of MICAL-1 +/+ or MICAL-1 −/− CA3 pyramidal neurons of culture experiments as shown in c . n >30 neurons per group of >3 independent cultures per genotype, from four to five different litters. Unpaired t -test, * P <0.05. Data are presented as means±s.e.m. ( c ) Dissociated P0–1 hippocampal cultures (HC) or co-cultures of P9 DG and CA3 neurons were fixed at 21 DIV and immunostained for SPO (red), vGlut1 (blue), CAMKII (not shown), Prox1 (not shown) and CTIP2 (not shown). Images show cell bodies of Prox1 − ;CTIP2 − CA3 pyramidal neurons. Mossy fibre synapses appear purple. Scale bar, 10 μm. ( d ) Multiple large, complex spines are extending from the somata of CA3 pyramidal neurons in adult MICAL-1 −/− ;Thy1-GFP mice. Panel at the right shows higher magnification of boxed area in middle panel. Scale bar, 10 μm. ( e – g ) Immunoelectron micrographs of the SP of CA3 in SPO–DAB-stained sections from the hippocampus of adult MICAL-1 −/− mice. ( e ) SPO + mossy fibre terminals containing numerous synaptic vesicles (yellow arrows) are located around a CA3 pyramidal neuron cell body (outlined in light yellow). ( f ) SPO + terminals form synapse-like junctions on a CA3 pyramidal neuron cell body (outlined in light yellow). Red arrows point to postsynaptic densities. ( g ) SPO + mossy fibre terminals contact a large and complex spine-like structure emanating from a CA3 pyramidal neuron cell body (outlined in light yellow). N, nucleus. Scale bars, 1 μm. Full size image The large number of ectopic synapses in MICAL-1 −/− mice raised the question of whether this phenotype reflects a role for MICAL-1 in mossy fibre synapse formation. We used the ‘synaptoporin (SPO) assay’ to adress this issue [32] . In this in vitro assay, punctate co-staining of SPO and vesicular glutamate transporter 1 (vGlut1) on Ca2+/calmodulin-dependent protein kinase II (CAMKII) + dendrites specifically labels mossy fibre synapses between DG and CA3 neurons. Immunostaining of 21 DIV hippocampal cultures derived from MICAL-1 +/+ or MICAL-1 −/− pups revealed no differences in the total number of SPO + ;vGlut1 + puncta on the proximal dendrites of CAMKII + CA3 neurons ( Fig. 3b ; Supplementary Fig. 4d ). However, in line with the increase in mossy fibre synapses around CA3 neuron somata in MICAL-1 −/− mice in vivo , the number of SPO + ;vGlut1 + puncta on CA3 somata was increased in MICAL-1 −/− cultures, as compared with MICAL-1 +/+ cultures ( Fig. 3b,c ; P <0.05; unpaired t -test). A similar increase was detected in 21 DIV co-cultures of DG neurons from MICAL-1 −/− mice with CA3 neurons from MICAL-1 +/+ mice. MICAL-1 −/− DG neurons made significantly more synaptic contacts onto MICAL-1 +/+ CA3 somata as compared with MICAL-1 +/+ DG neurons ( Fig. 3b,c ; P <0.05; unpaired t -test). To confirm these findings and assess whether or not MICAL-1 is required in DG neurons in vivo to negatively regulate mossy fibre synapse formation in the SP, sections from MICAL-1 −/fl ; Rbp4-Cre and MICAL-1 +/+ ; Rbp4-Cre mice were immunostained with antibodies against SPO. In line with the results from the SPO culture assay, numerous SPO + puncta were observed in the SP of CA3 in MICAL-1 −/fl ; Rbp4-Cre but not MICAL-1 +/+ ; Rbp4-Cre mice ( Supplementary Fig. 4e ). Analysis of MICAL-1 +/+ ; Thy1-GFP (green fluorescent protein) and MICAL-1 −/− ; Thy1-GFP mice, in which DG granule cells and CA pyramidal neurons are sparsely labelled with GFP, revealed that large, complex spines were extending from the somata of MICAL-1 −/− but not MICAL-1 +/+ CA3 pyramidal neurons ( Fig. 3d ). Finally, we examined the ectopic synapses in the SP of MICAL-1 −/− mice in more detail by performing immunoelectron microscopy (EM) for SPO. Ultrastructural analysis revealed the presence of numerous SPO + mossy fibre terminals around CA3 pyramidal neuron somata in the SP of MICAL-1 −/− mice ( Fig. 3e ). These aberrantly located terminals formed synapse-like junctions containing numerous SPO + vesicles directly on the somata of CA3 pyramidal neurons ( Fig. 3f ) or on large and branched spine-like structures emanating from the soma, often forming multiple postsynaptic densities ( Fig. 3g ). Together, these results show that MICAL-1 is required in DG neurons to negatively regulate the formation of mossy fibres synapses at the somata of CA3 neurons. MICAL-1 regulates PSA-NCAM cell surface expression How does the intracellular protein MICAL-1 control the lamina-restricted projection of mossy fibres? Thus far, in vivo roles for MICAL proteins have only been established in Drosophila . Here, Mical binds to plexinA and functions as a unique actin-remodelling enzyme in plexin/semaphorin-mediated repulsive axon guidance [20] , [25] . In vertebrate species, MICALs specifically bind the vertebrate homologues of plexinA (plexinA1–A4) [33] . This is intriguing since vertebrate plexinAs have been implicated in shaping lamina-specific mossy fibre pathways. However, several observations suggest that the lamination defects observed in MICAL-1 −/− mice do not result from impaired plexinA signalling. First, while genetic ablation of plexinA2 and/or plexinA4 , but not other plexinAs, induces mossy fibre lamination defects [8] , [9] , [34] , [35] , [36] ( Supplementary Fig. 5a ), these defects are clearly distinct from those observed in MICAL-1 −/− mice ( Fig. 2 ). Second, in line with this dissimilarity, growth cone responsiveness of MICAL-1 −/− DG granule cells to two different plexinA4 ligands, Sema3A and Sema6A, is intact ( Supplementary Fig. 5b,c ). Third, several wiring defects previously reported in knockout mice for plexinAs or their ligands were not detected in MICAL-1 −/− mice ( Supplementary Figs 5d,6 ). To uncover the molecular mechanisms by which MICAL-1 sculpts mossy fibre connectivity, we next microdissected the infrapyramidal region by laser capture microscopy at P10–P11 and subjected the collected samples to mass spectrometry. The infrapyramidal region was selected because it contains mossy fibres of the IPB, which are severely disrupted in MICAL-1 −/− mice. Mass spectrometry identified 404 unique protein hits, and gene ontology (GO) analysis of these candidates revealed an enrichment for proteins involved in protein localization (such as Rab proteins) and cell projection organization ( Supplementary Table 2 ). Remarkably, genetic ablation of two proteins in these GO classes, that is, Rab GDP dissocation inhibitor-α and neural cell adhesion molecule (NCAM), had been reported previously to cause mossy fibre lamination defects that phenocopy those found in MICAL-1 −/− mice [11] , [37] . GDP dissocation inhibitor regulates the activity of small GTPases of the Rab family in vesicle fusion and intracellular trafficking and thereby controls the secretion and surface expression of various proteins, including cell adhesion and guidance molecules [38] . NCAM is a member of the immunoglobulin superfamily of cell adhesion molecules (IgCAMs) that mediates cell–cell interactions and has broad functions in axon growth and guidance [7] . These observations led us to test the idea that MICAL-1 regulates mossy fibre development by controlling the cell surface levels of NCAM. To test this hypothesis, we first examined the expression of NCAM in and on growth cones of cultured DG granule cells by immunocytochemistry. Several NCAM antibodies were tested but none yielded specific cell surface immunostaining patterns. We therefore used anti-polysialic acid (PSA)–NCAM antibodies. NCAM is one of the few proteins that is posttranslationally modified by the addition of PSA, and enzymatic or genetic ablation of PSA reveals that the mossy fibre lamination defects seen in NCAM −/− mice result from removal of polysialyated NCAM [39] , [40] . In line with our hypothesis, cell surface expression of PSA-NCAM was reduced on growth cones derived from MICAL-1 −/− DG neurons and intracellular expression of PSA-NCAM was increased and locally condensed ( Fig. 4a ). Quantification of PSA-NCAM expression confirmed this observation ( Fig. 4b ; P <0.05, P <0.001; unpaired t -test). These data show that MICAL-1 controls NCAM intra- and extracellular distribution. 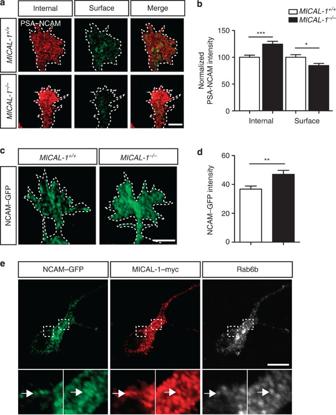Figure 4: Changes in the cell surface and intracellular expression of PSA–NCAM inMICAL-1-deficient growth cones. (a) Immunocytochemistry for PSA–NCAM on growth cones of 1 DIV DG granule cells obtained from P7 mice. Internal (red) and cell surface (green) pools of PSA–NCAM are visualized separately. Scale bar, 5 μm. (b) Fluorescent intensity of experiments as in (a) was quantified by measuring the surface and internal mean grey value for each growth cone. Surface levels were divided by internal levels per growth cone before normalization. All data were normalized to WT. +/+ 100 growth cones from 67 cells; −/− 116 growth cones from 68 cells, from three independent experiments. Unpairedt-test, *P<0.05, ***P<0.001. Data are presented as means±s.e.m. (c) Immunocytochemistry for GFP on growth cones of 2 DIV DG cultures transfected with NCAM–GFP cDNA. Scale bar, 5 μm. (d) Graph shows quantification of the intensity (mean grey value) of NCAM–GFP signals as shown in (c). +/+ 126 growth cones from 39 cells; −/− 107 growth cones from 33 cells, from three independent experiments. Unpairedt-test, **P<0.01. Data are presented as means±s.e.m. (e) Immunocytochemistry to detect GFP (NCAM), myc (MICAL-1) and endogenous Rab6b in transiently transfected 2 DIV hippocampal neurons from P0 WT mice. Boxed regions are shown at higher magnification at the bottom of each panel. White arrows indicate examples of vesicular structures containing MICAL-1–myc, NCAM–GFP and Rab6. Scale bar, 10 μm. Figure 4: Changes in the cell surface and intracellular expression of PSA–NCAM in MICAL-1 -deficient growth cones. ( a ) Immunocytochemistry for PSA–NCAM on growth cones of 1 DIV DG granule cells obtained from P7 mice. Internal (red) and cell surface (green) pools of PSA–NCAM are visualized separately. Scale bar, 5 μm. ( b ) Fluorescent intensity of experiments as in ( a ) was quantified by measuring the surface and internal mean grey value for each growth cone. Surface levels were divided by internal levels per growth cone before normalization. All data were normalized to WT. +/+ 100 growth cones from 67 cells; −/− 116 growth cones from 68 cells, from three independent experiments. Unpaired t -test, * P <0.05, *** P <0.001. Data are presented as means±s.e.m. ( c ) Immunocytochemistry for GFP on growth cones of 2 DIV DG cultures transfected with NCAM–GFP cDNA. Scale bar, 5 μm. ( d ) Graph shows quantification of the intensity (mean grey value) of NCAM–GFP signals as shown in ( c ). +/+ 126 growth cones from 39 cells; −/− 107 growth cones from 33 cells, from three independent experiments. Unpaired t -test, ** P <0.01. Data are presented as means±s.e.m. ( e ) Immunocytochemistry to detect GFP (NCAM), myc (MICAL-1) and endogenous Rab6b in transiently transfected 2 DIV hippocampal neurons from P0 WT mice. Boxed regions are shown at higher magnification at the bottom of each panel. White arrows indicate examples of vesicular structures containing MICAL-1–myc, NCAM–GFP and Rab6. Scale bar, 10 μm. Full size image Secretory vesicle accumulation in areas of abnormal F-actin The observation that MICAL-1 −/− growth cones display reduced cell surface expression, but enhanced and locally condensed intracellular expression of PSA-NCAM, supports the possibility that targeting of NCAM to the cell surface is perturbed in MICAL-1 −/− neurons. To test this idea, we transiently transfected dissociated hippocampal neurons with carboxy-terminally GFP-tagged NCAM. As reportedly previously, NCAM–GFP labelled the Golgi complex and vesicular structures in neurites and growth cones of WT neurons [41] ( Fig. 4c,d ). In MICAL-1 −/− neurons, GFP signals were increased and NCAM–GFP + vesicles accumulated in the central domain of the growth cone, in contrast to the more homogeneous NCAM–GFP + distribution observed in WT growth cones ( Fig. 4c ). Quantification of NCAM–GFP signals confirmed an increase in NCAM–GFP in MICAL-1 −/− growth cones ( Fig. 4d ; P <0.01; unpaired t -test). Taken together with the intracellular increased expression of endogenous PSA-NCAM in MICAL-1 −/− growth cones ( Fig. 4a,b ), this suggests that MICAL-1 is required for targeting NCAM to the membrane. Why does NCAM accumulate in MICAL-1 −/− growth cones? We have recently shown that MICAL-3 in HeLa cells serves as a molecular linker between Rab8A on Rab6 vesicles and ELKS at the plasma membrane during vesicle fusion [42] . Rab6 localizes to secretory (exocytotic) vesicles that are transported from the Golgi to the plasma membrane and that carry cargos for secretion or membrane insertion [42] , [43] . Defects in vesicle trafficking or fusion could explain the accumulation of NCAM in MICAL-1 −/− growth cones. To test a model in which MICAL-1 is involved in trafficking Rab6 vesicles containing NCAM, we first determined whether MICAL-1 and NCAM co-exist in Rab6 vesicles. Due to antibody incompatibilities, we used expression constructs for NCAM and MICAL-1 in combination with Rab6–GFP or Rab6 antibodies to co-localize these proteins. Transient transfection of NCAM–GFP and MICAL–myc in hippocampal neurons revealed co-localization of NCAM–GFP and MICAL-1 in vesicular structures ( Supplementary Fig. 7a ). This distribution pattern is in line with the normal vesicular distribution of endogenous MICAL-1 in the growth cones of young neurons ( Fig. 1d ). Similarly, transfection of MICAL–myc and Rab6–GFP confirmed the labelling of Rab6-positive vesicles by MICAL-1 ( Supplementary Fig. 7b ). Finally, transfection of MICAL–myc and NCAM–GFP, combined with immunocytochemistry for Rab6 revealed that NCAM and MICAL-1 co-exist in a subset of Rab6-decorated secretory vesicles ( Fig. 4e ). Together, these results suggest that the trafficking of Rab6 vesicles that contain NCAM may be perturbed in MICAL-1 −/− embryos. To test this idea, we generated mouse embryonic fibroblasts (MEFs) from MICAL-1 +/+ and MICAL-1 −/− embryos and stained these cells for endogenous Rab6. Although MEFs do not express NCAM, they represent an excellent cellular system for studying vesicle biology ( Supplementary Fig. 7c ). Whole-cell Rab6 density, excluding the Golgi area, was quantified, as well as the density of Rab6 vesicles in four randomly selected areas at the cell periphery. Although the overall density of Rab6 vesicles was unchanged in MICAL-1 −/− MEFs, as compared with control MEFs, the number of Rab6 vesicles at the cell periphery was significantly increased ( Fig. 5a,b ; P <0.0001; unpaired t -test). Furthermore, many MICAL-1 −/− MEFs displayed a compact, round morphology, contrasting with their normal fibroblast-like irregular shape. Total cell area values obtained from analyses of whole-cell Rab6 density, showed that MICAL-1 −/− MEFs were significantly smaller as compared with control cells ( Fig. 5a,b ; P <0.001; unpaired t -test). Since the abnormal morphology of MICAL-1 −/− MEFs hinted at cytoskeletal changes, we next assessed F-actin distribution. In MICAL-1 −/− MEFs, F-actin appeared strongly bundled and the amount of peripheral F-actin was increased ( Fig. 5a,b ; P <0.0001; unpaired t -test). Interestingly, the vast majority of Rab6 vesicles at the cell periphery in MICAL-1 −/− MEFs accumulated in dense F-actin bundles ( Fig. 5a ). 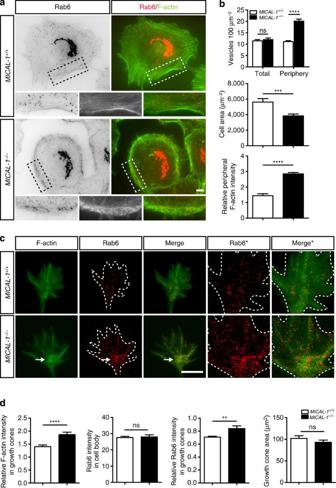Figure 5: Secretory vesicles accumulate in abnormal F-actin-rich regions ofMICAL-1−/−growth cones. (a) Immunofluorescent staining for Rab6 (red) together with phalloidin staining (green) in MEFs. Panels on the left show inverted contrast images of the Rab6 staining. Higher magnifications are derived from the boxed areas. Scale bar, 10 μm. (b) Quantification of the number of Rab6 vesicles 100 μm−2, MEF cell area and the intensity ratio between staining for F-actin at the cell periphery and in the central domain of the cell. MEFs were used at passage number 6. Rab6 data was obtained from 15 WT and 15 knockout MEFs, peripheral F-actin was calculated from seven WT and nine knockout MEFs. Area was measured from 19 WT and 22 KO MEFs. Unpairedt-test, ***P<0.001, ****P<0.0001. Data are presented as means±s.e.m. (c) Immunofluorescent staining for Rab6 (red) together with phalloidin staining (green) in growth cones of mouse DG neuron cultures. Scale bar, 5 μm. (d) Quantification of the intensity of F-actin, Rab6 vesicles in the cell body and the growth cone (relative to the cell body), and growth cone area. Obtained from 79 growth cones from 57MICAL-1+/+cells and 88 growth cones from 58MICAL-1−/−cells of individual experiments. **P<0.01, ****P<0.0001, unpairedt-test. Data are presented as means±s.e.m. Figure 5: Secretory vesicles accumulate in abnormal F-actin-rich regions of MICAL-1 −/− growth cones. ( a ) Immunofluorescent staining for Rab6 (red) together with phalloidin staining (green) in MEFs. Panels on the left show inverted contrast images of the Rab6 staining. Higher magnifications are derived from the boxed areas. Scale bar, 10 μm. ( b ) Quantification of the number of Rab6 vesicles 100 μm − 2 , MEF cell area and the intensity ratio between staining for F-actin at the cell periphery and in the central domain of the cell. MEFs were used at passage number 6. Rab6 data was obtained from 15 WT and 15 knockout MEFs, peripheral F-actin was calculated from seven WT and nine knockout MEFs. Area was measured from 19 WT and 22 KO MEFs. Unpaired t -test, *** P <0.001, **** P <0.0001. Data are presented as means±s.e.m. ( c ) Immunofluorescent staining for Rab6 (red) together with phalloidin staining (green) in growth cones of mouse DG neuron cultures. Scale bar, 5 μm. ( d ) Quantification of the intensity of F-actin, Rab6 vesicles in the cell body and the growth cone (relative to the cell body), and growth cone area. Obtained from 79 growth cones from 57 MICAL-1 +/+ cells and 88 growth cones from 58 MICAL-1 −/− cells of individual experiments. ** P <0.01, **** P <0.0001, unpaired t -test. Data are presented as means±s.e.m. Full size image To examine whether similar defects are present in neurons, Rab6 and F-actin were visualized in dissociated DG neuron cultures at 1 DIV. Using these cultures, growth cone area was determined and Rab6 and F-actin intensities were quantified throughout the entire growth cone or cell body of each neuron. In line with our observations in knockout MEFs, an increase in F-actin was observed in the central domain of MICAL-1 −/− growth cones and in large bundles emanating from this region towards the growth cone membrane. In addition, the number of Rab6 vesicles in the growth cone was increased in MICAL-1 −/− neurons, as compared with control, and many vesicles accumulated in areas of abnormal F-actin expression ( Fig. 5c,d ; P <0.001, P <0.0001; unpaired t -test). No changes were observed in the size or shape of MICAL-1 −/− growth cones, nor in the intensity of Rab6 immunostaining in the cell body ( Fig. 5d ). Thus, Rab6 secretory vesicles, which contain MICAL-1 and NCAM, accumulate in regions of abnormally organized actin in MICAL-1 −/− growth cones. MICAL-1 redox regulation of F-actin and secretory vesicles We have recently shown that MICAL-3 serves as a molecular linker between Rab8A on Rab6 vesicles and ELKS at the plasma membrane during vesicle fusion [42] . Defects in vesicle fusion could explain the accumulation of vesicles in MICAL-1 −/− growth cones. However, in contrast to MICAL-3, MICAL-1 binds Rab8A but not ELKS [42] , [44] , [45] . Since MICAL-1 can form oligomers (unpublished observations), we explored the possibility that MICAL-1 heterodimerizes with MICAL-3 to gain access to ELKS and regulate vesicle fusion. However, whereas co-immunoprecipitation experiments confirmed the previously established interaction between MICAL-1 and NDR1 (nuclear Dbf2-related) [46] , no binding between MICAL-1 and MICAL-3 was observed ( Fig. 6a,b ). Consistent with this observation no recruitment of MICAL-1–GFP to membrane regions expressing exogenous mCherry–MICAL-3 or nCherry–ELKS was observed in HeLa cells using total internal reflection fluorescence microscopy ( Supplementary Fig. 8a,b ). These results, coupled with our observation that MICAL-1 is not visibly enriched at the plasma membrane, argue against a prominent role for MICAL-1 as a molecular linker during vesicle docking or fusion. 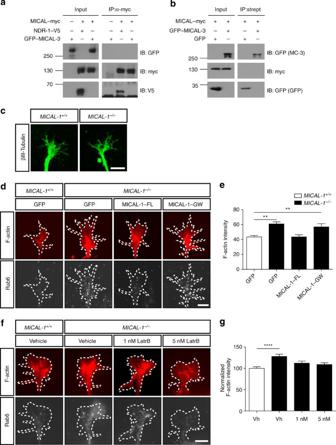Figure 6: Interdependent regulation of the actin cytoskeleton and vesicle distribution in the growth cone by MICAL-1 redox activity. (a) IP of myc-tagged MICAL-1 from HEK293 cells. Immunoblots were probed with the indicated antibodies: GFP (MICAL-3), myc (MICAL-1) and V5 (NDR1). Full-size western blots can be found inSupplementary Fig. 9. (b) Biotin–streptavidin pulldown of MICAL-3 from HEK293 cells. Immunoblots were probed with the indicated antibodies: GFP (MICAL-3, upper panel; and GFP control, lower panel) and myc (MICAL-1). IB: immunoblot; IP: immunoprecipitation; numbers indicate protein size in kDa. (c) Immunofluorescent staining for βIII-tubulin in growth cones of mouse hippocampal cultures derived fromMICAL-1+/+orMICAL-1−/−pups. Scale bar, 5 μm. (d) Immunofluorescent staining for Rab6 (white) together with phalloidin staining (red) in growth cones of mouse hippocampal cultures derived fromMICAL-1+/+orMICAL-1−/−pups transfected with the indicated constructs. FL WT; GW, enzymatically inactive MO domain. Scale bar, 5 μm. (e) Quantification of the intensity of F-actin in growth cones as ind. WT GFP,n=19; KO GFP,n=50; KO FL,n=27; KO GW,n=30 growth cones. One-way ANOVA, **P<0.01. Data are presented as means±s.e.m. (f) Immunofluorescent staining of F-actin and Rab6 following treatment with vehicle (Vh), 1 or 5 nM latrunculin B for 1 min. Scale bar, 5 μm. (g) Quantification of the intensity of F-actin in growth cones as inf. WT Vh,n=111; KO Vh,n=91; KO 1 nM,n=87; KO 5 nM,n=123 growth cones from three individual experiments. Data are normalized on WT vh. One-way ANOVA, ****P<0.0001. Data are presented as means±s.e.m. Vh, vehicle. Figure 6: Interdependent regulation of the actin cytoskeleton and vesicle distribution in the growth cone by MICAL-1 redox activity. ( a ) IP of myc-tagged MICAL-1 from HEK293 cells. Immunoblots were probed with the indicated antibodies: GFP (MICAL-3), myc (MICAL-1) and V5 (NDR1). Full-size western blots can be found in Supplementary Fig. 9 . ( b ) Biotin–streptavidin pulldown of MICAL-3 from HEK293 cells. Immunoblots were probed with the indicated antibodies: GFP (MICAL-3, upper panel; and GFP control, lower panel) and myc (MICAL-1). IB: immunoblot; IP: immunoprecipitation; numbers indicate protein size in kDa. ( c ) Immunofluorescent staining for βIII-tubulin in growth cones of mouse hippocampal cultures derived from MICAL-1 +/+ or MICAL-1 −/− pups. Scale bar, 5 μm. ( d ) Immunofluorescent staining for Rab6 (white) together with phalloidin staining (red) in growth cones of mouse hippocampal cultures derived from MICAL-1 +/+ or MICAL-1 −/− pups transfected with the indicated constructs. FL WT; GW, enzymatically inactive MO domain. Scale bar, 5 μm. ( e ) Quantification of the intensity of F-actin in growth cones as in d . WT GFP, n =19; KO GFP, n =50; KO FL, n =27; KO GW, n =30 growth cones. One-way ANOVA, ** P <0.01. Data are presented as means±s.e.m. ( f ) Immunofluorescent staining of F-actin and Rab6 following treatment with vehicle (Vh), 1 or 5 nM latrunculin B for 1 min. Scale bar, 5 μm. ( g ) Quantification of the intensity of F-actin in growth cones as in f . WT Vh, n =111; KO Vh, n =91; KO 1 nM, n =87; KO 5 nM, n =123 growth cones from three individual experiments. Data are normalized on WT vh. One-way ANOVA, **** P <0.0001. Data are presented as means±s.e.m. Vh, vehicle. Full size image MICALs were recently identified as organizers of the actin cytoskeleton that oxidize actin through their amino-terminal MO domain thereby decreasing the amount of actin polymerization in Drosophila [21] , [23] . Our findings support and extend these data by showing that loss of MICAL-1 causes an increase in F-actin in vertebrate neurons. Another cytoskeletal target of MICAL-1, the microtubule cytoskeleton [47] , appeared intact in MICAL-1 −/− neurons ( Fig. 6c ). The observation that Rab6 secretory vesicles accumulate in regions of MICAL-1 −/− growth cones that display aberrant F-actin organization is noteworthy since the actin cytoskeleton regulates multiple, distinct aspects of vesicle targeting in neurons [48] . To determine whether or not the MO domain is implicated in mediating the cytoskeletal and vesicle defects observed in MICAL-1 −/− growth cones, we next performed rescue experiments by transfecting WT and MICAL-1 −/− hippocampal neurons with DNA constructs encoding for GFP, full-length MICAL-1 (MICAL-1–FL) or a FL MICAL-1 protein with an enzymatically inactive MO domain (MICAL-1–GW) [22] , [47] . Exogenous expression of MICAL-1 in MICAL-1 −/− growth cones normalized F-actin levels and vesicle distribution, while locally enhanced F-actin and accumulated vesicles were observed in MICAL-1 −/− growth cones transfected with MICAL-1–GW mutant or with GFP, as a control ( Fig. 6d,e ; P <0.01, one-way ANOVA). No effects of GFP or MICAL-1 proteins were observed in WT growth cones. These data are compatible with a model in which MICAL-1 redox activity organizes the actin cytoskeleton and thereby the distribution of secretory vesicles. To provide further and more direct support for this model, we treated dissociated cultures with latrunculin B, an actin-depolymerizing agent, and assessed the distributions of F-actin and Rab6 vesicles. We first determined that treatment of WT growth cones with 1 or 5 nM latrunculin B for 1 min induced a mild decrease in F-actin, while leaving growth cone morphology intact. As expected, latrunculin B treatment reduced the levels of abnormal F-actin in the central region of MICAL-1 −/− growth cones and concomitantly normalized the distribution of Rab6 vesicles ( Fig. 6f,g ; P <0.0001, one-way ANOVA). Taken together, these results suggest that MICAL-1 expressed on vesicles, or in other parts of the growth cone, regulates the actin cytoskeleton and thereby modulates the trafficking of Rab6 secretory vesicles containing NCAM. MICAL-1 regulates the cell surface levels of IgCAMs in vivo Our data show that MICAL-1 controls the cell surface expression of PSA-NCAM in vitro . To address whether MICAL-1 serves a similar role in vivo , hippocampal sections were immunostained for PSA-NCAM or close homologue of L1 (CHL1) in the presence or absence of detergent to reveal cell surface versus total protein expression. CHL1, an IgCAM related to NCAM [7] , was included because CHL1 −/− and MICAL-1 −/− mice display highly similar mossy fibre defects [12] , [49] , [50] . PSA-NCAM and CHL1 were strongly expressed on mossy fibres in CA3 and no apparent differences in total PSA-NCAM and CHL1 immunostaining in the hippocampus were detected between MICAL-1 +/+ and MICAL-1 −/− mice with the exception of an aberrant localization of PSA-NCAM + and CHL1 + mossy fibres. In contrast, cell surface expression of both IgCAMs was reduced in MICAL-1 −/− mice ( Fig. 7a ). To further address this issue, NCAM and CHL1 levels were analysed in subcellular fractions of hippocampi from P10 MICAL-1 +/+ and MICAL-1 −/− mice. In each experiment, band intensity of cell surface protein signals was measured and normalized to a simultaneously detected loading control. In line with our immunohistochemical data, western blot analysis detected increased expression of NCAM and CHL1 in the cytoplasmic fraction (S3) and decreased expression in the membrane-enriched fraction (P3) of MICAL-1 −/− hippocampus, as compared with MICAL-1 +/+ mice. Total levels of NCAM and CHL1 in MICAL-1 −/− hippocampi were similar to control (H), indicating that MICAL-1 does not control the overall expression levels of these proteins. The subcellular expression of another IgCAM, L1, was similarly altered but subcellular expression of several unrelated proteins was unchanged ( Fig. 7b,c ). 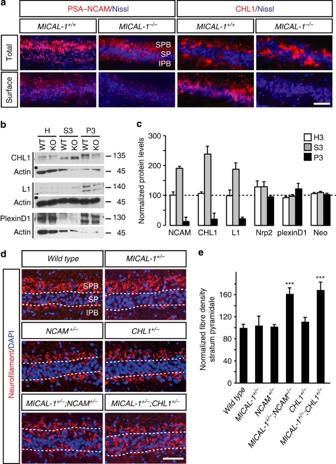Figure 7: MICAL-1 regulates IgCAM cell surface expression to control mossy fibre laminationin vivo. (a) Immunohistochemistry for PSA–NCAM or CHL1 in coronal sections of P55 mice. Staining was performed in the presence or absence of detergent to visualize total and cell surface expression, respectively. SP, stratum pyramidale.n=6MICAL-1+/+,n=5MICAL-1−/−. Scale bar, 90 μm. (b) Subcellular fractions of the hippocampus of P10 mice were subjected to western blot analysis using the indicated antibodies. Each experiment contained an internal loading control (actin). Representative examples are shown, full blots inSupplementary Fig. 9. Numbers at the right indicate kDa. H, homogenate; KO,MICAL-1knockout; P3, membrane; S3, cytosol; WT, wild type. (c) Quantification of band intensity of experiments as shown in (b) was performed by scanning densitometry. Signals were normalized to internal actin control and data were expressed as % of WT in each experiment. Graph shows means±s.e.m. from at least three independent experiments. Neo, neogenin; Nrp2, neuropilin-2. (d) Immunostaining of coronal sections of the hippocampus of P55 mice of the indicated genotypes using anti-NF antibodies (red) together with DAPI staining (blue). Scale bar, 140 μm. (e) Quantification of the genetic interactions between MICAL-1, NCAM and CHL1.n=5–7 mice for each genotype.P<0.001 compared with single heterozygous mice, one-way ANOVA. Data are presented as means±s.e.m. Figure 7: MICAL-1 regulates IgCAM cell surface expression to control mossy fibre lamination in vivo . ( a ) Immunohistochemistry for PSA–NCAM or CHL1 in coronal sections of P55 mice. Staining was performed in the presence or absence of detergent to visualize total and cell surface expression, respectively. SP, stratum pyramidale. n =6 MICAL-1 +/+ , n =5 MICAL-1 −/− . Scale bar, 90 μm. ( b ) Subcellular fractions of the hippocampus of P10 mice were subjected to western blot analysis using the indicated antibodies. Each experiment contained an internal loading control (actin). Representative examples are shown, full blots in Supplementary Fig. 9 . Numbers at the right indicate kDa. H, homogenate; KO, MICAL-1 knockout; P3, membrane; S3, cytosol; WT, wild type. ( c ) Quantification of band intensity of experiments as shown in ( b ) was performed by scanning densitometry. Signals were normalized to internal actin control and data were expressed as % of WT in each experiment. Graph shows means±s.e.m. from at least three independent experiments. Neo, neogenin; Nrp2, neuropilin-2. ( d ) Immunostaining of coronal sections of the hippocampus of P55 mice of the indicated genotypes using anti-NF antibodies (red) together with DAPI staining (blue). Scale bar, 140 μm. ( e ) Quantification of the genetic interactions between MICAL-1, NCAM and CHL1. n =5–7 mice for each genotype. P <0.001 compared with single heterozygous mice, one-way ANOVA. Data are presented as means±s.e.m. Full size image The mossy fibre defects observed in MICAL-1 −/− mice closely resemble those found in NCAM −/− and CHL1 −/− hippocampi. To further investigate whether or not MICAL-1 acts in concert with NCAM and CHL1 during mossy fibre pathfinding, we analysed single and compound heterozygous-mutant mice. Histological examination of MICAL-1 +/− , NCAM +/− and CHL1 +/− mice revealed no apparent mossy fibre lamination defects at P55 ( Fig. 7d ). However, transheterozygous MICAL-1 +/− ; NCAM +/− and MICAL-1 +/− ; CHL1 +/− mice exhibited a significant increase in the number of mossy fibres in the SP, as compared with WT ( Fig. 7e ; P <0.001; one-way ANOVA), phenocopying MICAL-1 −/− , NCAM −/− and CHL1 −/− single homozygous-null mutants. This robust genetic interaction in vivo , combined with our immunohistochemical, biochemical and in vitro data, show that MICAL-1, NCAM and CHL1 function in a common pathway to control the lamina-specific projection of mossy fibres. We report that MICAL-1 controls the growth cone membrane targeting of cell adhesion molecules (IgCAMs), through redox regulation of the actin cytoskeleton. This molecular mechanism dictates IgCAM cell surface levels and, as a result, the function of IgCAMs in the development of lamina-specific hippocampal mossy fibre connections ( Fig. 8 ). These findings for the first time establish an in vivo role for a vertebrate MICAL protein, and they provide insight into the poorly characterized molecular basis of lamina-specific neural circuit assembly. Further, they reveal mechanisms that control protein cell surface expression in neurons and unveil previously uncharacterized cellular functions for cytoskeletal regulation by MICAL proteins. Finally, our data show that MICALs can influence secretory vesicle behaviour not only through direct but also through indirect, actin-dependent, mechanisms. 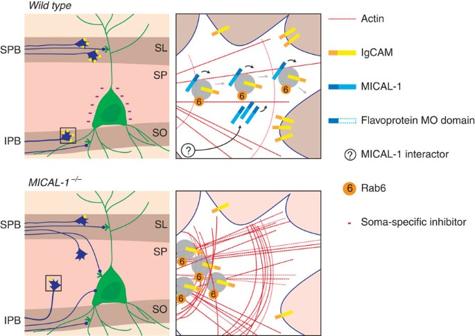Figure 8: MICAL-1 regulates IgCAM membrane targeting during hippocampal mossy fibre lamination. InMICAL-1−/−mice, secretory vesicles containing IgCAMs accumulate in the growth cone thereby preventing delivery of these proteins at the growth cone membrane. This results in lower IgCAM cell surface expression causing defects in the lamination of hippocampal mossy fibres and synapses. Thus, redox regulation of the cytoskeleton by MICAL-1 is critical for the proper membrane trafficking of cell surface proteins and thereby for lamina-specific neural circuit assembly. See text for details. Figure 8: MICAL-1 regulates IgCAM membrane targeting during hippocampal mossy fibre lamination. In MICAL-1 −/− mice, secretory vesicles containing IgCAMs accumulate in the growth cone thereby preventing delivery of these proteins at the growth cone membrane. This results in lower IgCAM cell surface expression causing defects in the lamination of hippocampal mossy fibres and synapses. Thus, redox regulation of the cytoskeleton by MICAL-1 is critical for the proper membrane trafficking of cell surface proteins and thereby for lamina-specific neural circuit assembly. See text for details. Full size image Inactivation of (PSA-)NCAM or CHL1 causes misrouting of mossy fibres due to defects in axon growth, fasiculation or synaptic pruning [11] , [12] , [39] , [49] , [50] . The mossy fibre defects found in MICAL-1 -mutant mice are remarkably similar to those observed following genetic or enzymatic inactivation of ( PSA-)NCAM or CHL1 and we observe robust genetic interactions between MICAL-1 +/− and NCAM +/− or CHL1 +/− mice. This together with reduced IgCAM cell surface expression on MICAL-1 −/− mossy fibres indicate that MICAL-1 is required to ensure appropriate IgCAM cell surface expression on mossy fibres and thereby regulates the lamina-restricted distribution of these axons ( Fig. 8 ). In line with the broad expression of MICAL-1 in the nervous system [30] , preliminary studies show additional defects in MICAL-1 −/− mice, such as changes in the size of specific cerebellar lobes and an enlarged ventricular system. Similar defects have been reported in NCAM −/− and CHL1 −/− mice [12] , [49] , [51] , supporting a more general role for MICAL-1-mediated IgCAM membrane targeting during neural development. Although MICALs have been implicated in semaphorin/plexinA signalling [22] , [33] , [47] , our present data do not support a role for MICAL-1 in plexinA-mediated mossy fibre pathfinding. It is, however, conceivable that the mossy fibre defects observed in plexinA −/− mice are MICAL dependent, but that absence of MICAL-1 in MICAL-1 −/− mice is compensated by MICAL-2 and/or MICAL-3. Future studies using mouse mutants lacking multiple MICAL genes are needed to address this issue. Although the SPB is shorter in MICAL-1 −/− mice and its lamination mildly disturbed, the IPB is much more severely affected in the absence of MICAL-1. The cause of this differential effect, which is also observed following inactivation of several other proteins that similar to MICAL-1 are expressed in IPB and SPB mossy fibres [49] , [52] , [53] , [54] , is unknown but may arise from differences in the origin, ontogeny and molecular makeup of the IPB and SPB. Typically, many types of cells are present within a target region, and axons form synapses with only a subset of them, often at specific domains of the target cell. Progress has been made in defining the mechanisms that determine synaptic specificity at the cellular level, but how subcellular synaptic specificity is achieved, particularly in the vertebrate nervous system, is less well-understood. Furthermore, studies so far have mainly focused on extracellular cues, while the intracellular determinants of these processes have remained largely unexplored [1] , [2] , [3] , [55] . Our data indicate that the redox protein MICAL-1 dictates subcellular specificity of DG–CA3 synapses via two distinct mechanisms. First, MICAL-1 restricts mossy fibres to the SL and stratum oriens, thereby confining these axons to the appropriate subcellular domains of CA3 pyramidal neurons: the proximal-most segments of their dendrites. Second, MICAL-1 controls the responsiveness of mossy fibres to unidentified soma-specific inhibitory signals on CA3 pyramidal neurons. This latter mechanism may act to control the transient innervation of the SP by mossy fibre collaterals during development [31] , [39] . Interestingly, PSA-NCAM has been reported to negatively regulate these transient innervations, either by promoting axon retraction or destabilizing transient synaptic contacts [39] . It is tempting to speculate that MICAL-1 regulates PSA-NCAM cell surface levels to negatively control the normally transient innervation of the SP. Alternatively, MICAL-1 may actively prevent axosomatic mossy fibre synapse formation, for example to direct synapses to proximal dendrites but not to adjacent somata of CA3 pyramidal neurons. Although further work is needed to address these models, our results provide insights into the poorly characterized intracellular mechanisms underlying subcellular synaptic specificity. Neural circuit assembly critically depends on precise spatiotemporal control of protein cell surface expression at the growth cone membrane. Although vesicular trafficking is an important mechanism to supply the membrane with new proteins, our understanding of how this process is regulated in neurons and how it functionally contributes to brain wiring is still limited [16] , [19] . Secretory vesicles that contain plasma membrane proteins are transported from the trans -Golgi network into growing neurites towards distant growth cones using the cytoskeleton as a scaffold. Our work uncovers an unexpected requirement for MICAL-1 in the distribution of secretory vesicles. Analysis of MICAL-1 −/− MEFs and DG neurons revealed a selective accumulation of Rab6 secretory vesicles. These vesicles contain NCAM in WT cells, while NCAM expression was decreased at the growth cone membrane in MICAL-1 −/− neurons, both in vitro and in vivo . These findings suggest that the supply of secretory vesicles containing NCAM to the growth cone membrane relies on MICAL-1. Interestingly, reduced cell surface expression of two other IgCAMs, CHL1 and L1, in MICAL-1 −/− hippocampi hints at a general role for MICAL-1 in the regulation of vesicles carrying IgCAMs. These effects are selective since the cell surface expression of proteins is normal in MICAL-1 −/− mice. Why do secretory vesicles accumulate in MICAL-1 −/− growth cones? The targeting of secretory vesicles to the plasma membrane is a complex multistep process, many aspects of which rely of precise spatiotemporal control of the actin cytoskeleton [48] , [56] , [57] . The increase in F-actin in the absence of MICAL-1, the apparent entrapment of vesicles in regions of abnormal F-actin, the ability of the actin-depolymerizing agent, latrunculin B, to dampen these defects, and the reported function of Mical as an F-actin disassembly factor through the post-translational oxidation of methionine 44 on actin [21] , [23] together support a model in which MICAL-1, through its MO domain, regulates F-actin dynamics, thereby influencing vesicle behaviour in the growth cone ( Fig. 8 ). These findings confirm and extend previous findings in Drosophila by showing that MICALs serve as enzymatic actin regulators in vertebrate neurons. Furthermore, they present physiological evidence of a role for MICAL redox activity in F-actin regulation, which had thus far largely relied on experiments using constitutively active MICAL constructs [21] , [23] , [27] , [58] , [59] . In addition, these data show that regulation of the cytoskeleton by MICALs functions in cellular processes other than axon repulsion and cell shape control. We have recently shown that another vertebrate MICAL, MICAL-3, links Rab6 vesicles to ELKS and thereby regulates their fusion in HeLa cells in an actin-independent manner [42] . Our results suggest that MICAL-1 serves a different role by acting through the cytoskeleton, providing support to the notion that individual MICAL proteins can use different molecular strategies to influence secretory vesicle behaviour. Interestingly, vesicles not only utilize, but can also modify, the actin cytoskeleton en route to their destination [60] . Since our data suggest that MICAL-1 may be present on vesicles but also binds other proteins known to reside in the growth cone, such as CasL, CRMP and plexins [25] , further work is needed to localize the precise site of MICAL-1 action. This may also help to establish which portion(s) of the vesicle’s route to the membrane is controlled by MICAL-1-mediated cytoskeletal control. Finally, it is possible that MICAL-1 impacts several different, and perhaps actin-independent, aspects of vesicle behaviour since it can bind different Rab proteins [25] , [44] , [61] . This idea is supported by studies showing that MICAL-like proteins, which resemble MICALs but lack the MO domain, control the recycling of cell surface proteins in epithelial cells [62] , [63] . However, no defects in IgCAM internalization or Rab11 vesicles were detected in MICAL-1 −/− growth cones (unpublished observations). Probing the extent to which MICAL-1 contributes to other aspects of neuronal vesicle biology will therefore require additional studies. In summary, we demonstrate that MICAL-1, through its effects on F-actin assembly, controls the intracellular distribution of secretory vesicles containing IgCAMs in neurons, thereby regulating the cell surface levels of these molecules and, as a result, their role in the development of lamina-restricted hippocampal connections. This intracellular control of protein cell surface expression adds another level of regulation to the control of lamina-specific connectivity and unveils unique molecular mechanisms that target neuronal membrane proteins. Interestingly, MICALs display a lamina-specific distribution in several brain regions other than the hippocampus (for example, in the cerebellum) and are also prominently expressed outside the nervous system. Therefore, MICAL-dependent strategies analogous to the one described here for mossy fibre lamination could be widely used to control developmental processes in diverse organ systems. Animals and tissue treatment All animal use and care was in accordance with institutional guidelines and approved by the animal experimentation committee (DEC). C57BL/6 mice were obtained from Charles River. Timed-pregnant, postnatal and adult mice were euthanized by means of cervical dislocation or an overdose of pentobarbital followed by transcardial perfusion. The morning on which a vaginal plug was detected was considered embryonic day 0.5 (E0.5) and the day of birth, postnatal day 0 (P0). Littermate controls were used, unless stated otherwise. For whole embryo staining, embryos (E10, E10.5, E11, E11.5 or E12.5) were collected in phosphate-buffered saline (PBS) and processed for immunohistochemistry with anti-NF antibodies (2H3). In brief, embryos were fixed in 4% paraformaldehyde (PFA) in PBS overnight at 4 °C, washed and incubated in 80% methanol. After inactivation of endogenous peroxidase activity, embryos were incubated with the 2H3 antibody in Tris-buffered saline (TBS) containing 5% skimmed milk, 5% DMSO and 1% Tween for 2 days at room temperature (RT). Then, embryos were incubated with horseradish peroxidase-coupled anti-mouse antibody and horseradish peroxidase activity was detected with 3,3′-diaminobenzidine (DAB) [64] . For in situ hybridization and section binding experiments, brains were directly frozen in 2-methylbutane (Merck). For immunohistochemistry, embryos and the brains of P0–P5 pups were collected in PBS and fixed by immersion for 0.5–6 h in 4% PFA in PBS at 4 °C. Postnatal (P5 onwards) and adult mice were transcardially perfused with ice-cold saline followed by 4% PFA and postfixed for 2 h. Samples were washed in PBS and cryoprotected in 30% sucrose. Brains were frozen in M-1 embedding matrix (Thermo Fisher Scientific) in 2-methylbutane and stored at −80 °C. Cryostat sections were cut at 16–20 μm, mounted on Superfrost Plus slides (Thermo Fisher Scientific), air-dried and stored desiccated at −20 °C. Generation MICAL-1- deficient mice A BAC containing a 5′ portion of the mouse MICAL-1 gene was obtained from Invitrogen (ResGen). BAC DNA fragments and a neomycin/FRT/loxP cassette (kindly provided by R.L. Huganir, Johns Hopkins School of Medicine, USA) were used to generate a conditional MICAL-1- targeting vector [65] . Following electroporation of the MICAL-1 -based targeting vector, targeted 129-derived ES clones were identified by Southern blot and injected into C57BL/6 blastocysts. Resulting male chimaeras were bred to C57BL/6 females to generate heterozygous mice carrying the mutation. MICAL-1 −/− and MICAL-1 fl/fl mice were obtained by crossing F1 heterozygous mice with mice that express Cre recombinase or FLP recombinase, respectively, in the germ cell lineage. The resulting lines were then moved into a C57BL/6 background (Charles River) by more than 10 successive backcrosses. To obtain DG-specific knockout of MICAL-1 , MICAL-1 fl/fl mice were crossed with BAC transgenic mice expressing Cre recombinase under the control of Rbp4 or POMC promotor sequences (Kindly provided by T.J. McHugh (RIKEN, Japan) and MMRRC, respectively) [66] . Rbp4-Cre and POMC-Cre mice were crossed with ROSA26;eYFP mice [67] to examine Cre recombination patterns in the hippocampus. MICAL-1 +/− mice were also crossed with NCAM +/− or CHL1 +/− mice [12] , [68] to obtain MICAL-1 +/− ; NCAM +/− and MICAL-1 +/− ; CHL1 +/− mice and littermate controls. Western blot analysis using a C-terminal anti-mouse MICAL-1 antibody [46] ( Supplementary Table 3 ) confirmed the lack of MICAL-1 protein in brain lysates of P5 MICAL-1 −/− mice. For PCR genotyping of the various mouse lines used in this study, see Supplementary Table 4 . Immunohistochemistry Sections were fixed for 1 h at RT, washed three times in TBS-T, blocked in TBS-T containing 0.2% bovine serum albumin (BSA) for 2 h at RT and incubated with primary antibodies overnight at 4 °C. After three washes in TBS, sections were incubated with the appropriate secondary antibodies diluted in TBS-T containing 0.2% BSA, for 1 h at RT. Then, sections were washed three times in TBS and coverslipped (for AlexaFluor antibodies), or incubated with avidin–biotin–peroxidase complex (Vectastain ABC kit; Vector Laboratories) in TBS containing 0.25% gelatin and 0.5% Triton X-100 for 1 h at RT. After two washes in TBS and a brief wash in 50 mM Tris–HCl, pH 7.6, sections were reacted with a solution containing 0.035% DAB and 0.015% hydrogen peroxide in 50 mM Tris–HCl for 15 min at RT. The reaction was terminated by several washes in 50 mM Tris–HCl and sections were mounted in glycerol [69] , [70] . Sections incubated with AlexaFluor antibodies were counterstained with either fluorescent Nissl (NeuroTrace; Invitrogen) or 4′,6-diamidino-2-phenylindole (DAPI) (Sigma), washed extensively in PBS and embedded in 90% glycerol. Staining was visualized using epifluorescent illumination on a Zeiss Axioskop A1 or by confocal laser scanning microscopy (Olympus FV1000). DAB-stained sections were dehydrated, cleared and coverslipped in Entellan (Merck). Staining was visualized using brightfield illumination on a Zeiss Axioskop A1. An antibody recognizing PSA-NCAM was used for NCAM staining, due to lack of NCAM antibodies suitable for cell surface staining. For more details on immunohistochemical procedures and quantification, Timm staining and EM, see Supplementary Methods . Tissue culture To obtain DG granule cell cultures, the hippocampus was dissected from P7–P9 brains (obtained from MICAL-1 +/− crosses or MICAL-1 +/+ and MICAL-1 −/− crosses) and cut into 350 μm slices using a tissue chopper (McIllwain). Subsequently, the DG was dissected from the slices. DG tissue was collected in 1 × Krebs medium (0.7% NaCl, 0.04% KCl, 0.02% KH 2 PO4, 0.2% NaHCO 3 , 0.25% glucose and 0.001% phenol red) and dissociated by incubation with 0.25% trypsin in Krebs/EDTA for 15 min at 37 °C. The reaction was halted by adding 2 mg soybean trypsin inhibitor, followed by trituration with a fire-polished Pasteur pipette in Krebs medium containing 2 mg soybean trypsin inhibitor and 20 μg ml − 1 DNAseI. Dissociated cells were resuspended in neurobasal medium supplemented with B-27, L -glutamine, penicillin/streptomycin and β-mercaptoethanol and plated onto poly- D -lysine- (PDL; 20 μg ml − 1 ) and laminin (40 μg ml − 1 )-coated glass coverslips in 24 well plates in a humidified incubator at 37 °C and 5% CO 2 . Medium was refreshed every other day by replacing half of the medium in each well with new medium. At the end of the experiment cultures were fixed by adding an equal volume of 8% PFA in PBS containing 8% sucrose (PFA-S) for 10–60 min at RT. To obtain mixed hippocampal cultures, the hippocampus was dissected from P0–P1 brains and collected in L15 dissection medium (Gibco) containing 7 mM HEPES (L15-HEPES). For dissociation, cells were incubated in 0.25% trypsin in L15-HEPES at 37 °C for 20 min, followed by trituration using a fire-polished Pasteur pipette in growth medium (Neurobasal medium supplemented with B-27, L-glutamine, penicillin/streptomycin and β-mercaptoethanol). Dissociated cells were resuspended in fresh growth medium and plated onto PDL- (20 μg ml − 1 ) and laminin- (40 μg ml − 1 ) coated glass coverslips. Medium was refreshed as described for DG cultures. Neuronal cultures were processed for immunocytochemistry using various antibodies. To visualize the microtubule cytoskeleton, primary hippocampal neurons were obtained from MICAL-1 +/+ or MICAL-1 −/− P0–P1 mice. At DIV1, cultures were shortly fixed in 4% PFA in PBS for 8 min, and immunostained with anti-βIII-tubulin antibodies. For the SPO assay, dissociated hippocampal cultures were generated from P0–P1 mice (obtained from MICAL-1 +/+ and MICAL-1 −/− crosses) and fixed at 21 DIV [32] . Alternatively, dissociated co-cultures were made from P9 MICAL-1 −/− DG neurons combined with P9 MICAL-1 +/+ CA3 neurons and from P9 MICAL-1 −/− DG neurons combined with P9 MICAL-1 +/+ CA3 neurons, and fixed at 21 DIV. Cultures were immunostained with primary antibodies against CamKII, VGlut1, SPO, Prox1 and CTIP2. CAMKII labels the dendrites of neurons, SPO and VGlut1 label synapses, Prox1 and CTIP2 label DG and CA1 neurons, respectively. For SPO analysis, confocal stacks were collected and images were corrected for background by adjusting intensity levels. Settings were saved so that the same confocal and analysis settings were used for every image. Analysis was done on cells without Prox1 or CTIP2 staining, to select CA3 neurons only. SPO + and VGlut1 + synapses were quantified using the Analyse Particle function from ImageJ. Dendritic length was quantified by semimanual tracing using the NeuronJ plugin in ImageJ. Puncta on cell soma were separated from puncta on dendrites. Data were expressed as puncta per μm (dendrites), or puncta per μm 2 (somata). Unpaired t -tests were performed using GraphPad Prism version 5.00 for Windows (GraphPad Software, San Diego, CA, USA, www.graphpad.com ). To visualize cell surface expression and the internal pool of endogenous PSA–NCAM or CHL1 in growth cones, dissociated DG neurons obtained from P7–9 WT and knockout mice (from MICAL-1 +/− crosses) were used. Cell surface molecules were labelled with anti-PSA–NCAM or anti-CHL1 antibodies at 1 DIV for 10 min at 37 °C and 5% CO2 in a humidified chamber. Then, neurons were carefully washed with warm PBS and fixed in warm 4% PFA in PBS containing 10% sucrose for 1 h. Cell surface PSA–NCAM or CHL1 was labelled with the appropriate Alexa 488-conjugated secondary antibodies diluted in PBS supplemented with 3% normal horse serum and 0.1% BSA. Subsequently, neurons were fixed for 8 min in 4% PFA at RT and permeabilized by incubation with blocking buffer containing 3% normal horse serum, 0.1% BSA and 0.1% Triton X-100 in PBS. The internal pool of PSA–NCAM molecules was labelled with newly diluted primary antibodies in blocking buffer and stained with Alexa 594-conjugated secondary antibodies. F-actin was stained with Alexa 350-conjugated phalloidin. Slides were mounted with Prolong Gold antifade (Invitrogen) and confocal stacks were collected with identical settings for each image. Fluorescent intensity was quantified in ImageJ by measuring the surface and internal mean grey value for each growth cone and cell body. Internal levels of mutant mice were normalized to internal levels in corresponding WT controls. Values of surface PSA–NCAM intensity were first divided by internal intensity values per growth cone (to control for differences in PSA–NCAM expression per cell). A mean ratio was calculated from all corrected WT values per experiment and all WT and mutant corrected surface values were normalized using this mean value within each experiment. Normalized values from each growth cone were used to calculate an average. Unpaired t -tests were performed using GraphPad Prism software. To study the distribution of NCAM–GFP-positive vesicles in growth cones, dissociated hippocampal cultures were generated from P0–P1 pups obtained from MICAL-1 −/− and MICAL-1 +/+ crosses. NCAM–GFP was generated by PCR amplification of the mouse NCAM coding region followed by ligation into pEGFP-N3, resulting in C-terminally tagged NCAM. NCAM–GFP was transfected at 1 DIV using Lipofectamine 2000 (Invitrogen) following standard protocols. At 2 DIV, cultures were fixed by adding an equal volume of warm 8% PFA in PBS containing 20% sucrose for 1 h and immunostained with a primary antibody against GFP in addition to phalloidin and DAPI staining (Sigma). Images were taken using a Zeiss Axioskop 2, using identical settings for each image. The fluorescent intensity of the NCAM–GFP and phalloidin signals were quantified by determining mean grey values from transfected growth cones and cell bodies using ImageJ software. Unpaired t -tests were performed using GraphPad Prism software. To assess the expression of MICAL-1 and NCAM in Rab6 secretory vesicles, dissociated hippocampal cultures obtained from P0–P1 WT pups were used. Myc-tagged FL MICAL-1, NCAM–GFP and/or Rab6–GFP [42] , [46] were transfected into hippocampal neurons at 1 DIV using Lipofectamine 2000. At 2 DIV, neurons were fixed by adding an equal volume of warm 8% PFA in PBS containing 20% sucrose for 10 min at RT and immunostained with primary antibodies for myc, GFP and Rab6. Images were generated using confocal laser scanning microscopy (Olympus FV1000). To study the distribution of Rab6 and F-actin in growth cones, dissociated DG neurons from P7–9 WT and knockout pups (obtained from MICAL-1 +/− crosses) were used. At 1 DIV, neurons were fixed by adding an equal volume of warm 8% PFA in PBS containing 20% sucrose for 1 h at RT. Rab6 immunostaining and Alexa 488-conjugated phalloidin staining were performed using standard protocols and staining was visualized using confocal laser scanning microscopy (Olympus FV1000). ImageJ was used to determine growth cone area and Rab6 and F-actin signal intensities throughout the entire growth cone or cell body. Values from growth cone measurements were divided by values from cell bodies from the same neuron to control for differences in Rab6 and F-actin expression between cells. Data were statistically analysed by unpaired t -tests using GraphPad Prism software. To perform rescue experiments, MICAL-1 +/+ and MICAL-1 −/− hippocampal neurons were transfected at DIV1 with peGFP, pRK5–FL–WT–MICAL–myc [46] and pFLAG–FL–MICAL-1–GW (a kind gift from Prof. Hiroaki Miki, Osaka University). At DIV2, neurons were fixed with 4% PFA with 10% sucrose in PBS and stained for Rab6 and F-actin as described above. ImageJ was used to determine F-actin signal intensity throughout the entire growth cone. These data were statistically analysed by one-way ANOVA with GraphPad Prism software. For latrunculin B treatment, 1 nM or 5 nM latrunculin B (Cayman Chemicals) was applied for 1 min in the growth medium of DIV1 primary hippocampal neuronal cultures. Longer treatment with these concentrations of latrunculin B or short incubations with higher concentrations led to a disturbance of growth cone morphology. Cultures were fixed for 10 min immediately after treatment by adding 8% PFA in PBS containing 8% sucrose to the tissue culture medium in a 1:1 ratio (fixative:medium). Cultures were stained for Rab6 and phalloidin as described above. ImageJ was used to determine F-actin signal intensity throughout the entire growth cone. A mean was calculated from measurements from vehicle-treated WT cultures and all WT and mutant values were normalized using this mean value within each experiment. Normalized values from each growth cone were used to calculate an average. One-way ANOVA was performed with GraphPad Prism software. For growth cone collapse assays, DG explants were dissected from P2–3 mice obtained from MICAL-1 +/− crosses and cultured on glass coverslips coated with PDL and mouse laminin (10 μg ml −1 ; Invitrogen). A 1 DIV recombinant proteins (Sema3A-Fc, Sema6A-Fc or Fc, as a control (R&D)) were added to the cultures for 1 h at 37 °C. Cultures were fixed and processed for immunocytochemistry with βIII-tubulin antibodies and counterstained with phalloidin to assess growth cone morphology [9] . For the generation, use and analysis of MEFs, see Supplementary Methods . Laser dissection microscopy Sections of P8–P11 mouse brains were cut at 16 μm on a cryostat and dried within the cryostat chamber to prevent protein degradation and were stored at −80 o C until use. Before the laser dissection procedure, sections were incubated in ice-cold 70% ethanol for 2 min and stained for 1 min with 1% (w/v) cresyl violet in 50% ethanol. Next, sections were washed briefly in ice-cold 70% ethanol and 100% ethanol and subsequently air-dried. Laser capture microdissection was performed on a PALM laser microscope system (Zeiss). The infrapyramidal region was isolated from both hippocampi from 68 sections per animal ( n =2) and laser catapulted into AdhesiveCap 200 opaque tubes (Zeiss). Dissected tissue was collected in lysis buffer (20 mM Tris pH7.5, 150 mM NaCl, 10% glycerol, 1% NP-40) containing protease inhibitor cocktail (Complete; Roche). After the procedure, LDS sample buffer (NuPAGE) and 2-mercaptoethanol were added and samples were stored at −80 °C. Samples were subjected to SDS–PAGE and Coomassie staining and gels were sent for mass spectrometry analysis at the Erasmus Proteomics Center (Rotterdam). The list of protein hits was cleaned for doubles and common contaminants such as keratin and abundant household proteins such as acetyl coenzyme A. Then, GO analysis Gene Ontology (version 1.2, 11/11/2012) was performed using WebGestalt2 ( http://bioinfo.vanderbilt.edu/webgestalt/ ) with a hypergeometric test, a significance level of 0.001 and at least two proteins per category. Subcellular fractionation Subcellular fractions were prepared from P10 hippocampus. For each independent experiment, hippocampi were isolated from eight MICAL-1 +/+ or eight MICAL-1 −/− mice and pooled per genotype. Three volumes of sucrose buffer (0.25 M sucrose, 1 mM EDTA, 5 mM NaCl, 10 mM KCl, protease inhibitor cocktail (Sigma) and 10 mM Tris–HCl pH7.5) were added, followed by homogenization using a 2 ml Wheaton tissue grinder (this homogenate fraction is H). The homogenate was centrifuged for at 800 g for 3 min at 4 °C to spin down the nuclei (resulting pellet is P1). The supernatant (S1) was transferred into another tube and centrifuged at 9,200 g for 10 min, to obtain a crude synaptic fraction (P2). The supernatant after this centrifuge step is S2. The S2 fraction was centrifuged at 165,000 g for 1 h, to acquire a cytosol-enriched fraction (supernatant, S3) and a plasma membrane-enriched fraction (pellet, P3). Pellets (P1–P3) were washed and resuspended in 200 μl sucrose buffer and 15 μl of each fraction (H, S1–S3, P1–P3) was used for western blot analysis. The efficiency of the fractionation procedure was confirmed by western blot analysis using antibodies against c-Jun, Synaptotagmin, Connexin-43 and Myosin (data not shown). For the detection of different cell surface proteins in the H, P3 and S3 fractions antibodies against NCAM, CHL1, L1, Neogenin, Neuropilin and PlexinD1 were used. Blots were digitalized and quantified using ImageJ. In each experiment, the intensity of cell surface protein signals was normalized to a simultaneously detected actin loading control. For immunoprecipitation experiments and alkaline phosphatase section binding, see Supplementary Methods . Blinding methods To avoid observer bias, all quantitative measurements in this manuscript were assessed while being unaware of genotype or condition. During analysis, raw data were named in a descriptive way, without revealing experimental group information. (Fluorescent) microscopic imaging was always done with the same settings within experiments, and analysing techniques were standardized. A single person analysed all data obtained within the experiments. All experiments were replicated at least three times. How to cite this article : Van Battum, E. Y. et al. The intracellular redox protein MICAL-1 regulates the development of hippocampal mossy fibre connections. Nat. Commun. 5:4317 doi: 10.1038/ncomms5317 (2014).